Adaptive response to sociality and ecology drives the diversification of facial colour patterns in catarrhines The faces of Old World monkeys and apes (Catarrhini) exhibit every possible hue in the spectrum of mammal colours. Animal colouration experiences selection for communication, physiology and ecology; however, the relative importance of these factors in producing facial diversity in catarrhines is not known. Here we adopt a comparative approach to test whether facial traits have evolved in tandem with social, geographic and ecological pressures across four catarrhine radiations. Our analyses reveal the underlying correlates of two major axes in the evolution of facial diversity. Facial colour patterns are linked to social factors, such that gregarious and highly sympatric species have evolved more colours in their faces. Facial pigmentation tends to be dominated by ecological factors, and species living in tropical, densely forested and humid habitats in Africa have evolved darker faces. Thus, both sociality and ecology have played a role in producing the highest diversity of faces within mammals. Diversity in animal colouration reflects competing selective pressures for a multitude of fitness-relevant functions, including communication (for example, individual and species recognition, mate selection) and homeostasis (for example, thermoregulation, UV absorption or protection). The faces of Old World monkeys and apes (Catarrhini) exhibit almost every possible hue in the spectrum of mammalian colouration, and these colours are often combined to form remarkably complex facial patterns such as those seen in mandrills, guenons and mangabeys. Catarrhines likely constitute the most diverse assemblage of facial colour patterns within mammals. Studies at the species-level in this clade suggest that some of the diversities in facial colours and their patterns may serve in social communication and mate recognition [1] , [2] , [3] . Facial colour pattern diversity in primates might also be driven by ecological demands for thermoregulation or camouflage, as the evolution of body colours in mammals is tied to these functions [4] , [5] , [6] , [7] . Although explicit tests for a link between ecology and facial diversity in catarrhines are lacking, ecological factors significantly predict levels of facial diversity in Neotropical primates (Platyrrhini), which form the sister group to catarrhines. In platyrrhines, darker faces evolved in species living in regions occupied by forests, such as the Amazon [8] . Social factors also explain some aspects of platyrrhine facial diversity, with complex colour patterns tending to evolve in species that live in small social groups and in high levels of congeneric sympatry [8] . When compared with their Neotropical relatives, catarrhines exhibit much greater diversity of facial colour patterns, occupy larger extensions and diversity of habitats, and show more extreme variation in average group size [9] . It is currently not known whether the evolution of the remarkable facial diversity in catarrhines has been shaped by the same factors governing the evolution of facial colours in platyrrhines or coat colour in mammals in general. Here we clarify the bases of the diversity of facial colouration in Old World monkeys and apes by integrating an unprecedented data set on quantitative metrics of facial, social and ecological traits to answer two fundamental questions. First, is the macroevolution of facial colour patterns explained by sociality? As the recognition of an individual’s identity can be the first step leading to many social interactions, we test the hypothesis that increases in pressures for recognition, both at the individual and species levels, are related to the evolution of more complex facial colour patterns across species. Following principles of modularity [10] , [11] , faces with more complex colour patterns would provide templates in which individual parts (variational modules) of the pattern can more easily and independently vary among members of a social group, leading to intraspecific differences that can be used by other members for individual recognition. Additionally, individual parts of the pattern have the potential to evolve across species and increase interspecific diversity that can aid in species recognition, which would be especially important to avoid interbreeding in closely related, sympatric species. Combining these trends, we would expect pressures for recognition to result in the evolution of more complex facial patterns in species that live in relatively large social groups and in high degrees of sympatry with closely related species. Second, do ecological gradients explain the evolution of facial pigmentation? We test the hypothesis that, if facial colours are adaptive for functions such as concealment from predators, thermoregulation and reduction of solar glare, then the evolution of facial pigmentation would be linked to the species’ geographic distribution and habitat characteristics. Specifically, we predict species living in dense, tropical forest habitats to have evolved overall darker faces, in accordance with Gloger’s Rule [7] , which suggests that darker colouration would facilitate concealment from predators by matching the background provided by the relatively darker environments in the forest understory [7] , [12] , [13] , [14] , as well as aid in thermoregulation [15] . We also predict overall lighter facial colouration in species living in temperate and open, brighter habitats, mainly because of advantages for camouflage and cooling. Trends in the macroevolution of facial pigmentation should be more obvious across geographic areas with accentuated ecological gradients—for example, within the African continent, which spans from tropical forests to subtropical desert ecosystems. In general, we predict that strong ecological pressures within a particular habitat lead to less complex facial colour patterns, as the whole face would evolve to be darker or lighter. Combining this with our previous hypothesis, social and ecological pressures may act antagonistically with regard to the complexity of facial colour patterns. Our comparative analyses across the four catarrhine radiations demonstrate that, whereas the evolution of facial pigmentation is associated with ecological gradients, increasingly complex facial colour patterns evolved in clades with higher pressures for social recognition (that is, large social groups and high levels of congener sympatry). Therefore, the extraordinary facial diversity of catarrhine primates is linked to social and ecological factors acting along largely separate axes of facial phenotype. Catarrhine social and ecological diversity To address our questions, we adopted a comparative approach and analysed facial traits from 139 catarrhine species within phylogenetic and spatial frameworks. Catarrhines include four radiations that inhabit a wide range of ecosystems and have repeatedly evolved high degrees of sociality along with striking facial features and displays. The Cercopithecidae (Old World monkeys) are widely distributed from Gibraltar throughout Africa and, in a second disjoint distribution, throughout central and southeast Asia. Cercopithecidae is divided into two ecologically and morphologically distinct lineages, Colobinae (leaf monkeys, including African colobus monkeys, Asian langurs and odd-nosed monkeys) and Cercopithecinae (cheek-pouch monkeys, including baboons, guenons and vervet monkeys in Africa, and macaques in Asia, Gibraltar and northwest Africa). Cercopithecids include some of the most social catarrhine species (for example, Mandrillus sphinx , with hordes of 800+ individuals on record [16] ). The gibbons and siamangs of the SE Asian rainforests make up the Hylobatidae, characterized by more modestly sized groups and variable social dynamics that often include high degrees of pair-bonding [17] . Finally, Hominidae [18] comprises four extant genera of great apes (and Homo , which was excluded from our sample). The great apes natively occupy forests in Africa and Asia. Socially, hominids range from solitary to highly gregarious with variable social systems even within species [19] . They have been extensively studied in regards to their use of facial features and expressions during social interactions [20] , [21] , [22] , [23] . Facial colour pattern diversity is explained by sociality Taxonomically, we found cercopithecines to exhibit the highest and most diverse values of facial colour pattern complexity (FCPC, Fig. 1 ), followed by colobines, hylobatids and, lastly, hominids ( Figs 2 , 3 , Supplementary Data 1 ). Spatial phylogenetic comparative analysis of all catarrhine species revealed highly significant correlation between sociality and FCPC across Old World primates. Species living in larger groups have faces with more complex colour patterns than species living in smaller groups (spatial Phylogenetic Generalized Least Squares regression: PGLS, β =0.008±0.002, t =3.11, df=90, P =0.0025, R 2 =0.369). Facial colour patterns were also more complex in species experiencing higher number of sympatric congener species, independent of group size ( β =0.145±0.052, t =2.22, df=90, P =0.029, R 2 =0.369). The error structure for this regression model follows a phylogenetic rather than a spatial structure, with a relatively high proportion of the variation being independent from these factors ( λ ′=0.60, ϕ =0, γ =0.40). This indicates that FCPC patterns tend to reflect evolutionary history more than shared habitat and that there might be other, unmeasured factors driving the evolution of FCPC. Only the presence of congeneric species was correlated with FCPC; neither the average nor maximum area of overlap among sympatric congeners was significantly correlated with FCPC. 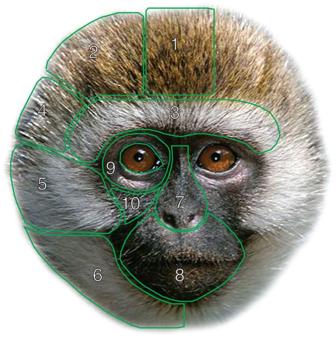Figure 1: The face of a vervet monkey illustrating the procedure used to characterize facial colour pattern complexity. Faces were subdivided into 10 areas that were used to record traits describing the hair and skin colour (1: Crown medial, 2: Crown lateral, 3: Forehead, 4: Margin dorsal, 5: Margin medial, 6: Margin ventral, 7: Nose, 8: Mouth, 9: Eye mask, 10: Cheek). Bilaterally symmetrical areas are shown for only one side of the face. Figure 1: The face of a vervet monkey illustrating the procedure used to characterize facial colour pattern complexity. Faces were subdivided into 10 areas that were used to record traits describing the hair and skin colour (1: Crown medial, 2: Crown lateral, 3: Forehead, 4: Margin dorsal, 5: Margin medial, 6: Margin ventral, 7: Nose, 8: Mouth, 9: Eye mask, 10: Cheek). Bilaterally symmetrical areas are shown for only one side of the face. 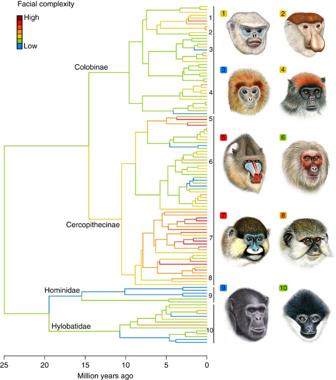Figure 2: Maximum-Likelihood ancestral state reconstruction of facial colour pattern complexity across catarrhine species. Warmer colours indicate more highly complex faces—that is faces in which the pattern is composed by many colours. Species shown in pictures are: (1)Rhinopithecus avunculus,(2)Nasalis larvatus,(3)Trachypithecus auratus,(4)Piliocolobus tephrosceles,(5)Mandrillus sphinx,(6)Macaca arctoides,(7)Cercopithecus cephus,(8)Miopithecus talapoin,(9)Pan troglodytesand (10)Nomascus leucogenys.Illustrations copyright 2012 Stephen D. Nash/IUCN/SSC Primate Specialist Group. Used with permission. Full size image Figure 2: Maximum-Likelihood ancestral state reconstruction of facial colour pattern complexity across catarrhine species. Warmer colours indicate more highly complex faces—that is faces in which the pattern is composed by many colours. Species shown in pictures are: (1) Rhinopithecus avunculus, (2) Nasalis larvatus, (3) Trachypithecus auratus, (4) Piliocolobus tephrosceles, (5) Mandrillus sphinx, (6) Macaca arctoides, (7) Cercopithecus cephus, (8) Miopithecus talapoin, (9) Pan troglodytes and (10) Nomascus leucogenys. Illustrations copyright 2012 Stephen D. Nash/IUCN/SSC Primate Specialist Group. Used with permission. 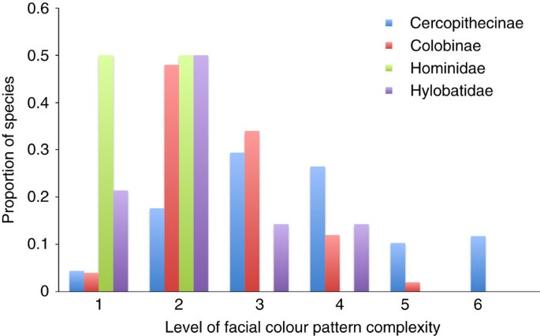Figure 3: Proportion of species within each catarrhine clade across levels of facial colour pattern complexity. Cercopithecid species (Cercopithecinae and Colobinae) score at the highest levels of complexity, hominids only rank at low levels of complexity and hylobatids have intermediate to low values (n=139 species). Full size image Figure 3: Proportion of species within each catarrhine clade across levels of facial colour pattern complexity. Cercopithecid species (Cercopithecinae and Colobinae) score at the highest levels of complexity, hominids only rank at low levels of complexity and hylobatids have intermediate to low values ( n =139 species). Full size image The relationships between FCPC and social factors for all catarrhines did not hold within each of the four major catarrhine radiations. Notably, some of these trends lost significance within the Cercopithecinae and Hylobatidae ( Table 1 ). In the former group, there is a significant interaction term between social group size and sympatry so that cercopithecines that live in large groups also live in low degrees of sympatry ( Table 1 ). The link between sympatry and FCPC was not tested in hominids, as the species’ ranges in our data set did not overlap among congeners. Table 1 Relationships between facial colour pattern complexity and social factors within catarrhine groups. Full size table Pigmentation trends are explained by ecological gradients Interspecific differences in pigmentation across most facial regions were significantly related to the species’ geographic distribution and ecological factors in their habitats ( Table 2 ; Fig. 4 ). Species living at lower, tropical latitudes, East of the Prime Meridian and in environments with a denser forest canopy have evolved darker facial parts and an overall darker face, whereas species living at higher, temperate latitudes and in western open environments have evolved more lightly coloured faces (spatial PGLS for average facial darkness: latitude (absolute value) β =−0.067±0.018, P =0.0008; longitude β =−0.030±0.017, P =0.103; canopy density β =0.016±0.006, P =0.009; mean temperature β =0.006±0.019, P =0.728; all df=107; λ ′=0.56, ϕ =0.27, γ =0.17; R 2 =0.13; Table 2 ). Across spatial PGLS regressions involving facial pigmentation of individual facial regions versus ecological variables ( Table 2 ), the values of ϕ ranged from 0.08 to 0.72 and λ ′=0.22–0.77 ( λ ′> ϕ in all cases), indicating a variable contribution of spatial versus phylogenetic effects across these traits. When the pigmentation data were analysed by continent, the trends were significant in African but not in Asian species ( Table 2 ; Fig. 4 ). In all cases, there was neither a clear relationship between facial pigmentation and average temperature across all species nor between FCPC and any ecological or geographic variable. Table 2 Major statistical trends in the evolution of facial pigmentation with respect to geographic and ecological variables. 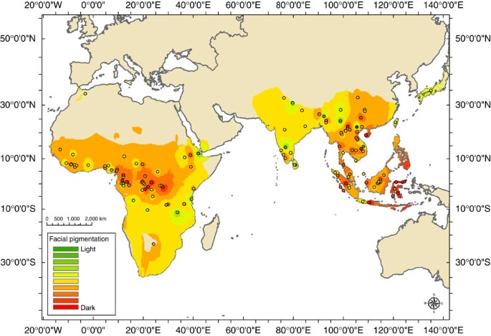Figure 4: Average darkness of catarrhine faces across their geographic range. Gradients were calculated via a cell moving window average based upon data on the centroid of the species’ geographic ranges (each indicated by a circle) and range overlap. Warmer colours illustrate areas occupied by species with overall darker faces. Full size table Figure 4: Average darkness of catarrhine faces across their geographic range. Gradients were calculated via a cell moving window average based upon data on the centroid of the species’ geographic ranges (each indicated by a circle) and range overlap. Warmer colours illustrate areas occupied by species with overall darker faces. Full size image Several lines of evidence suggest that facial `cues' are crucial to social communication across primates. Beyond the striking diversity of their faces, primates have intricate and highly conserved neurological pathways for facial recognition [24] , [25] , [26] , [27] , and multiple species have evolved conspicuous facial colours that function during mate selection (for example, red [28] , [29] ). In the New World primate radiation (Platyrrhini), the evolution of facial colour patterns is linked to social recognition; species with small social groups have evolved complexly patterned faces [8] . The results presented here expand upon this finding by confirming that facial diversity in catarrhines also evolved in tandem with social group size. However, diversity trends in catarrhines are the opposite from platyrrhines; highly gregarious catarrhines have evolved more complexly patterned faces. The divergent trends between platyrrhines and catarrhines may be explained by a higher reliance on facial expressions and displays for intraspecific communication in catarrhines [30] , [31] , [32] , [33] , [34] . For example, guenons ( Cercopithecus spp.) present complex facial colour patterns that are further advertised through stereotyped head ‘flagging’ movements during courtship or appeasement behaviours [3] , [31] . Thus, more complex faces could have evolved along with an increased ability for facial displays as a strategy to enhance individual recognition in larger groups. Differences in habitat use by platyrrhines versus catarrhines may also have a role, as visibility of facial cues is likely to be affected by the amount of clutter in the habitat and the distances among social group members. Quantitative data on the use of facial expressions [30] , [35] , and their relation to metrics of habitat use and social system, are crucial to test these hypotheses. Across all primates studied to date, higher levels of sympatry with closely related species are associated with the evolution of more complexly patterned faces. Higher facial colour complexity may be a path to achieve phenotypes that are unique and more easily recognizable in the context of multiple sympatric congeneric species. As these species share an ancestral facial template and, in this case, the same habitat, changing the colour of individual patches is a way of generating facial differences without fully compromising functional demands imposed by the environment (see below). The evolution of higher facial colour complexity within genera indicates de-coupling of the phenotype of different facial regions, which is consistent with the idea that these might constitute variational modules [10] . Modularity of the primate face is a likely advantage of these more structured facial colour patterns because it can enable higher levels of interspecific diversity [10] , [36] , [37] that would in turn be beneficial for species recognition. A modular framework characterizes the cranial morphology of many mammals, including primates [38] , [39] , [40] ; however, facial colour patterns have not been investigated in the context of modularity even though research suggests that various aspects of this system might be modular. First, work on mammal and insect colour patterns indicates that there is modular genetic control to the presence of colour patches and types of colouration [41] , [42] . Second, primate studies propose that some neurological elements in the process of face recognition are specific to certain functions, thus modular in that sense [43] . Further studies, in particular of the ontogeny of facial colour patterns, are necessary to further understand the modular structure of colour patches in primate faces. Intra- and interspecific social functions seem to be the major drivers of the evolution of FCPC; however, colour shading is tightly linked to spatial and ecological factors. Consistent with findings on the evolution of body colour in primates [14] , the pigmentation of most facial regions shows patterns that suggest adaptive evolution to habitat. Darker, melanin-based colours in the face and body [14] have evolved in tropical, more densely forested regions where these colours may reduce predation pressure by making individuals more cryptic to visually oriented predators [12] and increase resistance against pathogens [44] . Arguments for selection of darker colours for protection against high levels of UV radiation [15] or for thermoregulation [45] are contentious because arboreal primates can exploit their habitat in three dimensions, and there has been little quantification of the proportion of time different species spend at different forest strata (for example, the upper canopy, which has the highest UV levels, versus the middle- and lower canopy, which are highly shaded [9] ). Interestingly, ecological trends in facial pigmentation are only observed for African species even though this involves a paraphyletic grouping of the species that live in this continent (Cercopithecinae, Colobinae and Hominidae each has representatives in both Africa and Asia). This highlights the key differences in the evolution of primate faces in Africa and Asia. Whereas there are much more distinct habitat gradients within the African continent, the archipelagic nature of some primate ranges in SE Asia may enable other factors (genetic drift, geographic isolation and habitat heterogeneity) to influence the evolution of facial colours in Asian species. Primate faces are astonishingly diverse. For the largest and most widespread of all primate radiations, we show that the evolution of facial diversity is significantly correlated with both ecological and social factors. Whereas facial pigmentation has evolved in tandem with environmental conditions, the macroevolution of facial colour patterns is strongly associated with social situations that demand enhanced recognition and varied communication. This work demonstrates how high levels of interspecific phenotypic diversity may arise to meet diverse functions and highlights the potential of modular structures in generating this diversity. Taxonomic sample Our analyses included four radiations within Catarrhini (Old World monkeys and apes, Supplementary Data 1 ): Cercopithecidae, which comprises a diverse array of African and Asian species ( N =119 species; 69 cercopithecines and 50 colobines); Hylobatidae, which includes the gibbons in Asia ( N =14 species); and Hominidae, for which we only included the great apes ( N =6 species). We did not include Homo sapiens in our analyses because of the species’ worldwide distribution and high intraspecific phenotypic variation, leading to problematic assignment of morphological, social and ecological data. Facial variables Facial colour patterns and pigmentation data were generated from photographs of adult males in the All the World’s Primate Database ( http://www.awpdb.com ) and Arkive ( http://www.arkive.org ). Samples per species included two to ten high-resolution close-up photographs, taken in the wild or in captivity. Facial colour patterns were quantified using the FCPC metric [8] . This measure represents the total number of uniquely different colour areas on the face. FCPC is calculated by subdividing the face into differently coloured areas ( Fig. 1 ) spanning the diversity in patterns across species and recording the colour of each area based on a reference scale [8] . All observations were made by one person (S.E.S.). Recording the colour of each facial area also allowed the assignment of a darkness score to each facial part (lowest values=white hair or depigmented skin; highest values=black hair or hyperpigmented skin [8] ) and the generation of a metric that approximated the degree of pigmentation of each facial region. Pigmentation scores across all facial regions were averaged to test for general trends in facial colour; this average was used in the graphic representation shown in Fig. 4 . Social and ecological variables Average group size was used as a proxy for sociality, as these data can be collected from the literature for a large number of primate species. The mean community size was used for species presenting fission–fusion societies. Species distribution and sympatry data were generated from geographic distribution shapefiles downloaded from the International Union for the Conservation of Nature database [46] . These shapefiles contain each species’ known range, depicted as polygons where a species is widespread, or as points where there are isolated records. For each species, we used tools in ArcView (ESRI, USA) to determine the overlap in geographic ranges and to generate data on the number of sympatric species at the genus level and the average area (in m 2 ) of these overlaps. Areas of overlap were converted to Logs 10 prior to analyses. ArcView was also used to generate data summarizing the species’ geographic ranges by calculating the centroid of each polygon and noting its latitude and longitude. The location of these centroids was restricted to be placed in landmasses. Absolute values of centroid latitudes were used for regressions (below), so that greater values represented ranges away from the Equator. Longitude values were not transformed. Raw centroid locations of species distribution were used to source data on canopy density, mean precipitation and average temperature for each species from the USGS Global Forest Resources Assessment data set (http://edc2.usgs.gov/glcc/fao) and the WorldClim Database [47] . Species were also classified by continent to investigate whether there were differences in the evolutionary trends between African and Asian species, as distribution ranges in these two continents are disjointed and span different magnitudes of environmental gradients. Phylogenetic and spatial analyses Phenotypic traits result from both selection for ecological adaptation and past evolutionary history; thus, comparative methods are necessary to disentangle the roles of these processes and to correctly test for trait correlations in an evolutionary context [48] , [49] . We used the Freckleton and Jetz [47] procedure to simultaneously estimate and account for the spatial and phylogenetic components of trait evolution in our regression models (R code available from R.P. Freckleton upon request). Three parameters are estimated simultaneously in these models [48] : ϕ , which measures the relative contribution of phylogenetic and spatial effects and varies between 0 (only ‘phylogenetic effects’, the error structure of the models follows a phylogenetic rather than a spatial structure) and 1 (only ‘spatial effects’, the error structure of the models follows a spatial rather than a phylogenetic structure); λ ′, a spatially corrected version of Pagel’s λ [50] , which is calculated as λ ′=(1− ϕ ) λ and varies from 0 (trait values are independent of phylogeny) to 1 (trait values are structured according to a Brownian motion model of evolution) and γ, which represents the proportion of trait variation independent of both space and phylogeny and is calculated as (1− ϕ )(1− λ ). Parameter estimates were based on a distance matrix generated from latitudes and longitudes of centroids of species’ distribution, paired with a recent species-level phylogeny [51] . We conducted spatial Phylogenetic Generalized Least Squared (spatial PGLS) regressions with a Brownian motion model of evolution and estimated ϕ , λ ′ and γ within this context. Facial traits (FCPC, pigmentation per region, average pigmentation across the face) were used as response variables in separate regression models, whereas social (group size, number of sympatric species and area of sympatry at the genus level) and ecological (geographic distribution, canopy density and average temperature) variables were the predictors. We found that annual precipitation was positively and significantly correlated with canopy density in our data set ( β =0.036±0.008; t =4.654; P =2.59 × 10 −5 ); thus, we only included canopy density in our regressions. Upon graphic exploration of the data, two outlier nodes were removed from the data set prior to analyses ( Papio anubis-P. cynocephalus and Colobus polykomos-C. vellerosus ). Phylogenetic analyses were conducted in R [52] using functions in the APE [53] , GEIGER [54] and NMLE [55] packages, and those kindly provided by R.P. Freckleton for spatial PGLS. How to cite this article: Santana, SE. et al. Adaptive response to sociality and ecology drives the diversification of facial colour patterns in catarrhines. Nat. Commun. 4:2765 doi: 10.1038/ncomms3765 (2013).